Superconception in mammalian pregnancy can be detected and increases reproductive output per breeding season The concept of superfetation, a second conception during pregnancy, has been controversial for a long time. In this paper we use an experimental approach to demonstrate that female European brown hares ( Lepus europaeus ) frequently develop a second pregnancy while already pregnant and thereby increase their reproductive success. After a new, successful copulation, we confirmed additional ovulations before parturition in living, late-pregnant females by detecting a second set of fresh corpora lutea using high-resolution ultrasonography. The presence of early embryonic stages in the oviduct, demonstrated by oviduct flushing, next to fully developed fetuses in the uterus is best explained by passage of semen through the late-pregnant uterus; this was confirmed by paternity analysis using microsatellite profiling. Subsequent implantation occurred after parturition. This superfetation, categorized as superconception, significantly increased litter size and permitted females to produce up to 35.4% more offspring per breeding season. It is therefore most likely an evolutionary adaptation. How could a female become pregnant while she is still pregnant? And what is the benefit? In mammals, maternal provisioning includes the periods of intrauterine development and lactation. In short-lived mammals with early maturity and a short reproductive lifetime (often described as r-selected species) [1] , the number of reproductive cycles within a breeding period is usually considered to be maximized if the next fertilization follows immediately after parturition. In a polyoestrous seasonal breeder such as the European brown hare ( Lepus europaeus ), reproductive cycle length could be even further shortened if a new conception already occurred during an ongoing intact pregnancy, thereby increasing the potential reproductive output within a breeding period. A new conception during an intact pregnancy is defined as superfetation [2] and was first suggested for the hare by Aristotle [3] . For superfetation to be successful, there are several challenges to overcome, such as stimulation of ovulation during pregnancy, which should be physiologically suppressed [4] , passage of semen through an already occupied uterus, considered to be unfeasible and unsuccessful [5] , [6] , and possibly implantation of a second set of embryos next to already implanted fetuses in the uterus. The diagnosis of superfetation in any species therefore requires an experimental demonstration of ovulation and fertilization during an intact pregnancy, the presence of discordantly developed offspring within the reproductive tract of the mother under tightly controlled conditions and the tracking of the two pregnancies irrespective of the mechanism that permits the phenomenon to occur [2] . As this has always been difficult for methodological reasons, superfetation has been controversial since ancient times [2] , [3] . Historically, the presence of discordantly developed fetuses within a uterus [3] , [7] was usually discarded as evidence [2] , as other explanations were readily available [2] and the physiological requirements for superfetation unlikely to be met. The European brown hare is a strictly induced ovulator; stimulation by copulation is considered a necessity [7] . In this paper, we investigate whether successful prepartum conception in European brown hares really exists, how possible mechanisms might operate and how such superfetation affects female reproductive success. Using a captive colony and a stepwise experimental approach, we demonstrate that superfetation in European brown hares exists, can be diagnosed in living individuals, is a widespread, regular occurrence, requires a second copulation during the last phase of the ongoing pregnancy and is most likely achieved by passage of semen through the late-pregnant uterus. On the basis of our observations that superfetation increases litter size and reduces each reproductive cycle by 4 days, we discuss its evolutionary origin and conclude that superfetation in the European brown hare is an evolutionary adaptation to shift maternal care from the postpartum to the prepartum stage and thus move postpartum care towards a precocial mode. Detection of superfetation through breeding-pair management In a large-scale experiment in a captive population of European brown hares, we studied pregnant females over four consecutive breeding seasons (January to September). In three groups of females, different tactics of breeding management were used. Copulation activity was confirmed by video surveillance. Mean pregnancy lasted 41.9 ± 0.7 days ( n =24 females and 35 litters), as measured in breeding pairs in which the male was only present for 1 day to procreate the initial litter and then removed (group A 'conventional breeders'). In breeding pairs permanently housed together (group B 'permanent breeders'), copulations were frequently observed by video surveillance 3–4 days before parturition. Parturition of successive litters occurred after an interval of 38.4 ± 1.0 days ( n= 6 females and 18 litters) [2] , [8] , [9] . To exclude the possibility that group B males had escaped video surveillance and copulated after parturition and that gestation period in group B females was unusually variable, a third group of breeding pairs (group C 'temporary breeders') were housed together temporarily for (1) 1 initial day to allow copulation, and after pregnancy was confirmed (2) for 5 days from day 36 to 41 of gestation. The interbirth interval in temporary breeders was 38.1 ± 1.8 days ( n= 7 females and 11 litters). If the conception of a new litter only starts after parturition of the previous litter, the interval between successive litters (permanent and temporary breeders) should have the same duration as 'normal' pregnancies (conventional breeders). However, the observed differences between mean interbirth intervals of these groups were significant (Kruskal–Wallis test, H= 30.614, d.f.=3 including group D, see below, P <0.00001): the gestation period of conventional breeders was significantly longer than the interbirth interval of either permanent ( post hoc multiple comparisons, t= 6.258, P <0.00001) or temporary breeders ( t= 6.636, P <0.00001), whereas there was no difference between permanent and temporary breeders ( t= 0.010, P= 0.99). Hence, in permanent and temporary breeders, the conception must have taken place before delivery, and thus superfetation must have occurred. This was also supported by just considering those six females subjected to both conventional and permanent breeding regimes. Their pregnancy period during conventional breeding was significantly longer (42.0 ± 0.7 days, n= 13 litters) than their own interbirth intervals during permanent breeding (38.4 ± 1.0 days, n= 18 litters) (Wilcoxon signed-rank test, exact P= 0.031). Ultrasonographic detection of superfetation The first indicator of a pregnancy is the ultrasonographic detection of corpora lutea of pregnancy as early as on day 3 of gestation, verified by the detection of a live embryo at day 11 of gestation [10] . Ultrasonographic examinations around delivery date in permanent and temporary breeders demonstrated a new set of corpora lutea in late pregnant females near the active corpora lutea of the current pregnancy up to 2 days before delivery ( n= 9 females in 11 litters) and indicated prepartum conception ( Fig. 1 ). Ultrasonography is therefore the first reliable criterion to demonstrate a second conception and thus superfetation in a living, late-pregnant female. Subsequent early embryonic stages [10] of new pregnancies were diagnosed by ultrasonographic detection shortly after the birth of the previous litter ( n= 10 females in 23 litters) up to 4 days earlier than would have been possible had fertilization occurred after parturition. 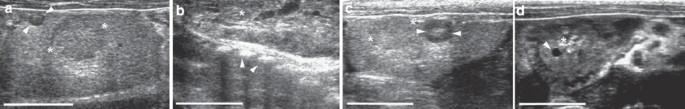Figure 1: Ultrasonographic detection of superfetation. (a) Late-pregnant females were ultrasonographically examined to detect a second set of new corpora lutea (white arrowheads), indicative of new ovulations during an ongoing gestation, next to the active corpora lutea (*) from the active pregnancy, in which (b) living fully developed fetuses are present inside the uterus (rib cage (white arrowheads) and part of thorax of a fully developed fetus next to placental tissue (*)). Frequent ultrasonographic examinations after delivery revealed (c) two sets of corpora lutea, the regressing ones from the previous pregnancy (*) and the now active ones (white arrowheads) from the gestation that resulted from superfetation, and (d) early embryonic structures (here, embryonic vesicles (white arrow heads) next to placental scars (*) from parturition 2 days ago), which were more developed than from fertilization after parturition would have been possible. The white size bar indicates 10 mm. Figure 1: Ultrasonographic detection of superfetation. ( a ) Late-pregnant females were ultrasonographically examined to detect a second set of new corpora lutea (white arrowheads), indicative of new ovulations during an ongoing gestation, next to the active corpora lutea (*) from the active pregnancy, in which ( b ) living fully developed fetuses are present inside the uterus (rib cage (white arrowheads) and part of thorax of a fully developed fetus next to placental tissue (*)). Frequent ultrasonographic examinations after delivery revealed ( c ) two sets of corpora lutea, the regressing ones from the previous pregnancy (*) and the now active ones (white arrowheads) from the gestation that resulted from superfetation, and ( d ) early embryonic structures (here, embryonic vesicles (white arrow heads) next to placental scars (*) from parturition 2 days ago), which were more developed than from fertilization after parturition would have been possible. The white size bar indicates 10 mm. Full size image Demonstration of two discordantly developed litters In six additional temporary breeding pairs, we studied the reproductive tract of the pregnant female after copulation with the male between days 36 and 41 of pregnancy in detail: we documented the presence of semen in a vaginal smear, demonstrated a new set of corpora lutea near the active corpora lutea of the current pregnancy by ultrasonography ( Fig. 1 ) and flushed the oviduct either before ( n= 2) or immediately after parturition ( n= 4) of the previous litter ( Supplementary Table S1 ). In all cases, the number of recovered embryos equalled the number of previously detected corpora lutea (Wilcoxon signed-rank test, exact P= 0.031). These methods directly confirmed the presence of early embryos in the oviduct coexisting with fully developed fetuses within the uterus ( Supplementary Fig. S1 ). Detection of embryonic loss and resorption Embryonic loss and resorption were diagnosed during ultrasonographic examinations of pregnant females. In a preimplantative stage up to day 5 of gestation, in which no embryonic structures can be ultrasonographically visualized [10] , no direct evidence for embryonic loss could be found. However, the number of expected embryos can be estimated from the number of corpora lutea detectable from day 3 of gestation onwards ( Fig. 2 ). Around implantation from days 6 to 10 of gestation, embryonic loss could be indirectly ascertained if fewer embryonic vesicles than corpora lutea were detected, as these represented the number of ovulations and hence the potential number of fertilized ova. Embryonic loss was also indirectly detected if the number of concepti declined in successive ultrasonographic examinations. After day 11 of gestation, the time when a living embryo can be first detected [10] , active processes of embryonic resorption could be visualized and followed up during the resorption process ( Fig. 2 ). In pregnancies with partial embryonic resorptions, a specific regression of some corpora lutea during gestation next to 'surviving' active corpora lutea was ultrasonographically observed according to the numbers of embryonic resorptions and fetuses developed to full term ( Fig. 2 ). Altogether, in 89 out of 159 pregnancies (56.0%) in 34 out of 45 females, embryonic loss occurred, that is, more ovulations were detected than offspring delivered. In 35 pregnancies, embryonic resorption was ultrasonographically detected by the visualization of a dead embryo and/or of the remaining extraembryonic structures ( Fig. 2 ). Embryonic death occurred until midpregnancy, a stage when organogenesis is nearly finished and the embryo itself is about 25 mm long [10] . The process of embryonic resorption was then ultrasonographically followed up until late pregnancy. Three litters were unusual in that they were conceived as a conventional pregnancy; yet, the size of the offspring varied substantially ( Supplementary Fig. S2 ). 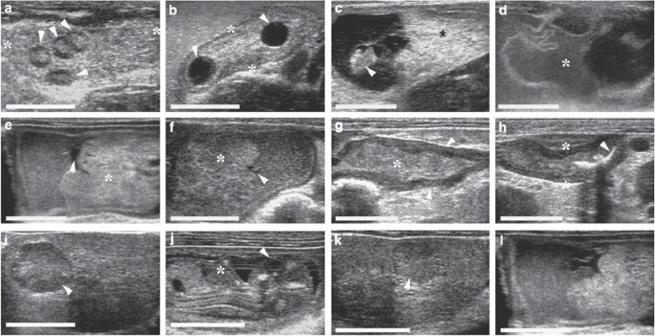Figure 2: Ultrasonographic detection of embryonic resorption. (a) In a preimplantative stage up to day 5 of gestation, the number of corpora lutea (white arrowheads), and hence the number of estimated embryos, can be counted. (b) Periimplantative (from days 6 to 10 of gestation), when embryonic vesicles can be seen but not yet a live embryo, the difference between the number of embryonic vesicles (white arrowheads) in the lumen of the uterus (*) and corpora lutea indicates early embryonic loss. (c–h) The direct ultrasonographic confirmation of postimplantative embryonic resorption can be carried out from day 11 of gestation onwards and typical stages of the course of embryonic resorptions can be visualized: (c) Loss of integrity: dead embryo (white arrowhead) but still intact placenta (*) and extraembryonic structures. (d) Embryo not detectable anymore and loss of integrity of extraembryonic structures (*). (e,f) Only small amounts of fluid remain (white arrowheads), decrease in size and compaction of resorption site, placental tissue (*) as the largest tissue part to be resorbed remains the longest. (g) Only undefined firm tissue (*) structures are left in the uterus (white arrowhead). (h) Last detectable stage of embryonic resorption: Scars (white arrowheads) from implantation in the endometrium of a uteruine loop (*). (i–l) Partial regression of corpora lutea according to partial embryonic resorptions: (i) active corpus luteum (white arrowhead) and (j) live embryo (eye (white arrowhead), heart (*)), (k) corpus luteum in regression (white arrowhead) and (l) resorption site. The white size bar indicates 10 mm. Figure 2: Ultrasonographic detection of embryonic resorption. ( a ) In a preimplantative stage up to day 5 of gestation, the number of corpora lutea (white arrowheads), and hence the number of estimated embryos, can be counted. ( b ) Periimplantative (from days 6 to 10 of gestation), when embryonic vesicles can be seen but not yet a live embryo, the difference between the number of embryonic vesicles (white arrowheads) in the lumen of the uterus (*) and corpora lutea indicates early embryonic loss. ( c – h ) The direct ultrasonographic confirmation of postimplantative embryonic resorption can be carried out from day 11 of gestation onwards and typical stages of the course of embryonic resorptions can be visualized: ( c ) Loss of integrity: dead embryo (white arrowhead) but still intact placenta (*) and extraembryonic structures. ( d ) Embryo not detectable anymore and loss of integrity of extraembryonic structures (*). ( e , f ) Only small amounts of fluid remain (white arrowheads), decrease in size and compaction of resorption site, placental tissue (*) as the largest tissue part to be resorbed remains the longest. ( g ) Only undefined firm tissue (*) structures are left in the uterus (white arrowhead). ( h ) Last detectable stage of embryonic resorption: Scars (white arrowheads) from implantation in the endometrium of a uteruine loop (*). ( i – l ) Partial regression of corpora lutea according to partial embryonic resorptions: ( i ) active corpus luteum (white arrowhead) and ( j ) live embryo (eye (white arrowhead), heart (*)), ( k ) corpus luteum in regression (white arrowhead) and ( l ) resorption site. The white size bar indicates 10 mm. Full size image Embryonic resorption also occurred in experimental groups. In breeding pairs permanently housed together (group B, n= 10 females and 27 cases), a subsequent pregnancy was diagnosed in 23 cases ( n= 7 females) shortly after the birth of the previous litter. Of these, five litters (21.8%) were completely resorbed, and 78.2% ( n= 18 litters in 6 females) were delivered. In temporary breeding pairs (group C), pregnancy did not develop if copulation did not occur during gestation. In those cases when it did ( n= 33 cases in 18 females), a second pregnancy was detected by ultrasonography; yet, in only 11 cases did the pregnancy come to full term (33%, n= 7 females). Experimental induction of superfetation In a fourth group (group D 'artificially inseminated breeders', n= 6 females), we successfully induced new pregnancies before delivery with artificial insemination [11] on day 38 of gestation in six out of nine (66.7 %) attempts, resulting in deliveries of a total of 19 leverets in six litters. The mean interval between births in pregnancies induced by artificial superfetation was 38.3 ± 1.3 days, not different from those of permanent breeders ( post hoc multiple comparison, t= 0.064, P= 0.95) or temporary breeders ( t= 0.111, P= 0.91), but significantly shorter than the gestation period of conventional breeders ( t= 6.813, P <0.00001). Testing the hypothesis of semen storage No pregnancy developed from artificial insemination at days 34 – 36 of gestation ( n= 12 attempts). Hence, the possibility of a successful induction of superfetation in European brown hares is restricted to the limited period of days 37 (minimum) to 41 of gestation [9] . We also examined whether superfetation requires copulation during this limited period of late-stage pregnancy simply to induce ovulation without actually siring the offspring. Fertilization would then occur via semen stored in the uterine folds from the earlier insemination [5] , [6] . This hypothesis predicts that copulation of pregnant females between days 36 and 41 of gestation (as documented by video surveillance) with vasectomized males—where libido is maintained but insemination of viable sperm averted—should result in a new conception (superfetation). Six different vasectomized males were mated with seven different females and ovulation was confirmed in all nine sterile matings through the ultrasonographic detection of corpora lutea, but no pregnancy ensued (Wilcoxon signed-rank test, exact P= 0.004). Paternity tests by microsatellite profiling revealed that in sequential matings of five different females with two males (altogether, eight different males, M#1 for induction of first pregnancy, M#2 for copulation during late pregnancy before birth), M#2 was the father of 17 of the 19 leverets in the five litters born from the second pregnancy (Wilcoxon signed-rank test, exact P <0.0001). In the two remaining offspring (from two different litters), their microsatellite profiles matched that of male M#2 but were not sufficiently unique to unambiguously exclude paternity of M#1 ( Supplementary Table S2 ). Detection of superfetation in a free-ranging population In our breeding colony, in 54.4% (37 out of 68) of the pregnancies when fertilization before delivery was possible, a new pregnancy and thus superfetation occurred, including 52.0% (13 out of 25) of the females ( Fig. 3 ). We then analysed an ultrasonographic data set obtained during a previous investigation of 143 living, free-ranging females [12] studied at different stages of pregnancy and for which gestational age was defined by applying established reference parameters [10] . In three out of seven late-pregnant females, in which we would expect superfetation to occur, small anechoic structures indicating new corpora lutea ( Fig. 4 ) were detected near the active corpora lutea of pregnancy. Hence, prepartum copulations and potential superfetation occurred in 42.9% of pregnancies in free-ranging females. This value is similar to the incidence of superfetation in our captive colony and the success in inducing artificial superfetation as described above (log likelihood ratio test, G= 0.93, d.f.=2, P= 0.63). 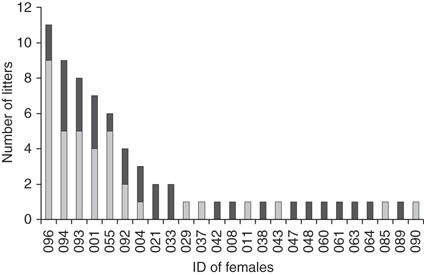Figure 3: Incidence of superfetation in the captive colony. In 68 pregnancies, superfetation was possible because of the presence of a fertile male with a late-pregnant female between days 36 and 41 of pregnancy. In 36 of these pregnancies and in 13 out of 25 females, a second pregnancy developed (superfetation) (light grey bars); in the other 32 pregnancies in 19 different females (dark grey bars), no further pregnancy developed. Of those females in which the opportunity for superfetation arose more than once, 7 out of 9 females (77.8%) had at least one pregnancy successfully conceived by superfetation. Figure 3: Incidence of superfetation in the captive colony. In 68 pregnancies, superfetation was possible because of the presence of a fertile male with a late-pregnant female between days 36 and 41 of pregnancy. In 36 of these pregnancies and in 13 out of 25 females, a second pregnancy developed (superfetation) (light grey bars); in the other 32 pregnancies in 19 different females (dark grey bars), no further pregnancy developed. Of those females in which the opportunity for superfetation arose more than once, 7 out of 9 females (77.8%) had at least one pregnancy successfully conceived by superfetation. 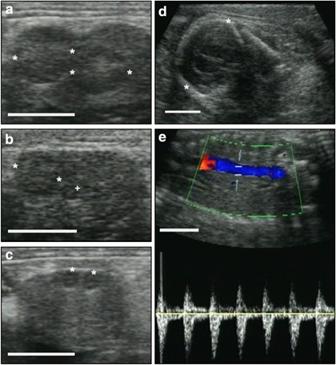Figure 4: Ultrasonographic diagnosis of prepartum ovulation in free-ranging individuals. (a) Section of left ovary with two corpora lutea of pregnancy (*). (b) Different section of left ovary with two different types of corpora lutea, one corpus luteum of pregnancy (*) 'belonging' to the fully developed first pregnancy, one small 'new' corpus luteum (+) from the second ovulation before parturition. (c) Section of right ovary with two small 'new' corpora lutea (*). (d) Section of the head (*) of a full-term fetus. (e) Doppler ultrasonogram indicating the heartbeat and liveliness of the full-term fetus and hence the demonstration of evidence for ovulations during an intact pregnancy in a free-ranging female. The white size bar indicates 10 mm. Full size image Figure 4: Ultrasonographic diagnosis of prepartum ovulation in free-ranging individuals. ( a ) Section of left ovary with two corpora lutea of pregnancy (*). ( b ) Different section of left ovary with two different types of corpora lutea, one corpus luteum of pregnancy (*) 'belonging' to the fully developed first pregnancy, one small 'new' corpus luteum (+) from the second ovulation before parturition. ( c ) Section of right ovary with two small 'new' corpora lutea (*). ( d ) Section of the head (*) of a full-term fetus. ( e ) Doppler ultrasonogram indicating the heartbeat and liveliness of the full-term fetus and hence the demonstration of evidence for ovulations during an intact pregnancy in a free-ranging female. The white size bar indicates 10 mm. Full size image Influence of superfetation on female reproductive output In our captive colony, the mean litter size at birth across the breeding season was 2.5 ± 1.2 (range 1–6, n= 131 litters, Supplementary Table S3 in which summaries of further parameters of reproductive output in relation to the mode of conception can be found). The average number of litters per season was 3.1 ± 0.5 (median=2.0, n= 41 females). The average number of reproductive seasons was 1.5 ± 0.1 (median=1.0); females produced up to six litters per year in up to four reproductive seasons. We used general linear mixed models (GLMMs) to test whether reproductive output depended on the mode of conception (without or with superfetation) while simultaneously checking for possible changes of reproductive output with litter order across the breeding season within a given year of reproduction (first, second (and so on) year of reproduction) or between breeding seasons across different years of reproduction for individual females. Changes in reproductive output with litter order might be expected because the first pregnancies of the year started in January and February; they were usually small and they could not have developed by superfetation ( Fig. 5 ). Data were available from a total of 131 litters from 41 females. Conception by superfetation significantly increased litter size by an average of 0.65 leverets (95% confidence interval 0.21–1.09; F 1,87 =8.92, P= 0.0037, Akaike Information Criterion (corrected)=344.93). Litter size also increased with litter order ( t= 2.531, d.f.=87, P= 0.013) by 0.08 leverets, with each order number within a given breeding season (95% confidence interval 0.017–0.14). Litter size did not depend on the year of reproduction ( t= 0.568, P= 0.57). In a GLMM for the number of corpora lutea per litter ( n =157 litters from 45 females, including cases in which no offspring were born), superfetation also increased the number of ovulations (ultrasonographically measured as number of corpora lutea) by an average of 0.58 corpora lutea, (95% confidence interval=0.13–1.02; F 1,109 =6.512, P= 0.012, Akaike Information Criterion (corrected)=526.44). The number of corpora lutea per litter also increased with litter order ( t= 3.71, d.f.=109, P= 0.00033) by 0.08 corpora lutea, with each order number within a given breeding season (95% confidence interval=0.055–0.18). The number of corpora lutea per litter declined with the year of reproduction ( t= 2.083, P= 0.04) by 0.32 corpora lutea (95% confidence interval 0.015–0.62). 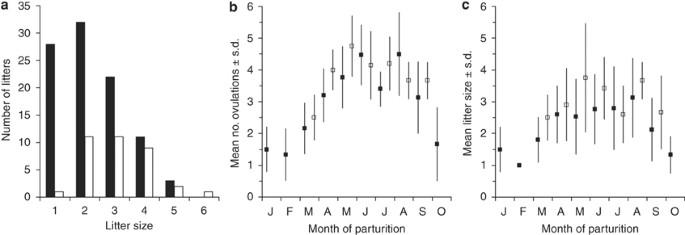Figure 5: Reproductive output with and without superfetation throughout the breeding season. (a) Frequency of litter sizes in relation to the mode of conception either conceived without (black bar) or with (white bars) superfetation. (b) Mean number of ovulations and (c) mean litter size of litters conceived without (black squares) or with (white squares) superfetation during the breeding season. Figure 5: Reproductive output with and without superfetation throughout the breeding season. ( a ) Frequency of litter sizes in relation to the mode of conception either conceived without (black bar) or with (white bars) superfetation. ( b ) Mean number of ovulations and ( c ) mean litter size of litters conceived without (black squares) or with (white squares) superfetation during the breeding season. Full size image With an increase in litter size, the expected reproductive output of a female using superfetation is potentially much higher than would be expected from merely shortening the interbirth intervals, as model calculations show ( Table 1 ). The expected reproductive output increases from 14.4 offspring per breeding season to 19.5, an increase by 35.4%. Table 1 The reproductive potential per breeding season of female European brown hares with and without superfetation. Full size table Consistent with the conventional definition of superfetation [2] , our results demonstrate that ovulations and fertilizations regularly occurred during established pregnancies in European brown hare females. They also imply that the mechanism of superfetation can overcome several substantial endocrine and potential immunological and microbial barriers. When superfetation occurs, two different sets of offspring are inside the reproductive tract of a female hare. The fully developed litter is present in the uterus, the early embryonic stages of the second litter conceived by superfetation is located in the oviducts. This explains why the subsequent second litter is not affected by the event of parturition. Hence, superfetation also implies the phenomenon of successful implantation of embryos early after parturition in an extensively burdened and destroyed uterine environment. Embryos or fetuses in the process of resorption create a discordant set of fetuses. Their appearance, however, was readily distinguished from the discordant shape of two sets of fetuses conceived by conventional pregnancy followed by superfetation. If fetuses in European brown hares in utero are discovered to be growth discordant, this is most likely a consequence of embryonic resorption or retardation but not of superfetation. As demonstrated by paternity analyses in the five pregnancies examined, superfetation in European brown hares is usually not achieved by semen stored from a previous copulation. The results also indicate that (1) copulation during late pregnancy is required for both ovulation and the delivery of fertilizing sperm and (2) semen must have passed the late-pregnant uterus for fertilization of a second set of ova during an established pregnancy. Hence, although the hypothesis of semen storage [5] , [6] cannot be completely rejected, it seems very unlikely under these conditions. Our results support the detailed findings of other authors with regard to evidence of superfetation in the European brown hare [2] . We have shown here that superfetation is used by many females. The prepartum conception also results in a shortening of the reproductive cycle and an increase in average litter size [8] , [9] , [13] . The relevance of possible superfetation for reproductive performance in wild populations had previously been doubted [14] , [15] , [16] . Our findings demonstrate that superfetation is found within free-ranging European brown hare populations and is not an artefact of captivity. The current sample size from the free-ranging population is too small to make a confident statement about the real incidence in natural populations, or to explore potential differences between populations. Yet, the observed incidence (three out of seven suitable females from the free-ranging population with evidence for superfetation) is similar to the incidence in captivity and stems from the height of the breeding season in April when such superfetation might routinely be expected. Excluding January and February, when the first pregnancy of the season occurred, the mean length of the remaining breeding season would be around 210 days. A comparison of the resulting expected reproductive output per female per season without and with superfetation shows that superfetation leads to a substantial increase of 35.4% ( Table 1 ). Superfetation can therefore produce a substantial increase in the reproductive output per female per breeding season. This suggests that—far from being a rare event—superfetation might be an evolutionary adaptation to enhance reproductive success and fitness of female European brown hares. We do not (yet) have sufficient data to assess postnatal development and survival to maturity of offspring conceived under conditions with and without superfetation, a common problem arising in studies evaluating the adaptive value of life history traits [17] . Superfetation should, however, be considered as an important part of a suite of reproductive traits that have favoured past and recent successful dispersal [18] and evolutionary and ecological success of the European brown hare [15] , [19] in comparison with other closely related species. The genus Lepus , or true hares, diverged from other members of the subfamily Leporinae, the rabbits, approximately 11.8 million years ago [20] . Rabbits exhibit a period of prolonged (altricial) postpartum parental care, whereas postpartum parental care in members of the genus Lepus is short (precocial). As in other species groups, the altricial mode is considered to be the ancestral one [21] , [22] . Precocial parental care and traits such as superfetation would then be derived characters. Among the members of the genus Lepus , gestation period can be variable. For instance, the snowshoe hare ( Lepus americanus ), basal in the phylogenetic tree of the Lepus spp . [20] , has a gestation period of 37 days [23] , which is shorter than that of the European brown hare (42 days). Nevertheless, up to that day of gestation, embryonic development is very similar [10] in both species. Thus, copulation on day 38 is a postpartum mating in the snowshoe hare and a mating during late pregnancy in the European brown hare. From this comparative developmental perspective, we suggest that superfetation has most likely evolved to suppress parturition during oestrus and to delay birth until the latest possible date before the implantation of the successive litter. In other words, superfetation would have been an additional tool in shifting parental care from the postpartum to the prepartum stage and thus further moved postpartum care towards a precocial mode. Within the classification scheme previously described [2] , superfetation in European brown hares should be categorized as superconception. Whether only European brown hares or also other members of the genus Lepus have evolved this mode remains to be determined. Study animals Data were collected from European brown hares kept under natural climatic conditions at the field research station of the IZW at 13° 50′ E and 52° 44′ N. Animals originally derived from a breeding colony in Nitra, Slovakia. The hares were housed in wooden pens (2×2 m 2 ) under natural climatic conditions. Food (modified rabbit pellets), fresh water and hay were always available ad libitum . Every cage was checked at least once a day. Young hares were weaned at 24 days postpartum and supplemented with oat flakes until 3 months of age. Cages consisted of two large compartments, each with one adult hare, which could be separated for purposes of breeding-pair management. Four cages were equipped with video cameras connected to a digital video recording device (VAS 2412-4 Q). This allowed 24 h monitoring of the breeding pairs for mating and parturition. Pregnancies were induced by natural mating with a fertile male ( n= 132) or through artificial insemination [11] ( n= 27). Day 1 of pregnancy was defined as the day of copulation, which was ascertained by breeding-pair management, artificial insemination [11] and/or video surveillance. The day when the newborn was found in the cage was noted as parturition date. For this purpose, cages were checked once a day starting 3 days before the predicted parturition date. Video surveillance showed that parturitions mainly happened in the period between late evening and early morning. Data from free-ranging animals were obtained in a previous study of the Leibniz Institute for Zoo and Wildlife Research on reproductive performance in European brown hares carried out in Germany between 1998 and 2003 [12] . Hares were caught in the field using nets and submitted to transabdominal ultrasonography as described below. Data were collected during the breeding season in February, April and June. The authors confirm that all experimental work on live animals complied with our institutional and governmental regulations. The institutes committee for animal welfare and ethics (letter 18.05.2005) and the Ministry for Agriculture, Environment and Consumer Protection (letter 06.07.2005) approved the experimental design in accordance with §8a of the German law of animal welfare (Tierschutzgesetz). Examinations of pregnancies We examined 159 pregnancies in 45 different females in four consecutive breeding seasons between 2004 and 2007. Owing to embryonic loss and resorptions, not all concepti detected by ultrasonography were brought to full term; 131 pregnancies in 41 different females finally led to the parturition of 325 offspring. All pregnant females were examined on a regular basis; altogether 486 examinations were performed using a standardized protocol, including a general health check, blood sampling, a complete transabdominal ultrasonographic evaluation of the reproductive tract [10] , [11] and weighing. Hares were caught in wooden boxes attached to the pen. Examinations were performed either under general anaesthesia or without anaesthesia using a specially prepared and appropriately sized wooden restraint box. For general anaesthesia, isoflurane (2.5 vol%, Isoba, Essex) and oxygen (1.5–2.0 l min −1 ) were applied with an inhalation mask. The hares were positioned in dorsal recumbency and the abdomen was manually shaved. Ultrasound transmission gel in combination with 70% alcohol was used to ensure optimal coupling during ultrasonographic examination. All ultrasound examinations were conducted with a real-time, B-mode scanning system (Diasus, Dynamic Imaging). This high-resolution ultrasound unit was equipped with four different linear ultrasound probes (5–10, 8–16, 10–22 and 16–28 MHz) and permitted the identification of structures down to the minimum size of 0.05 mm. Images were recorded on the internal hard drive and a Mini DV recording unit (GV-D 900/E, Sony) connected to a S-VHS port for further evaluation. During transabdominal ultrasonography, the general developmental status and the quantity and quality of structures were evaluated and documented. Then, the number of ovulations was ascertained by the number of corpora lutea detected. For this purpose, both ovaries were sequentially imaged from left to right and from cranial to caudal for a complete coverage. Follicles and corpora lutea were counted, measured and their position documented. With this method it was possible to follow the development of single functional structures, especially corpora lutea, during repeated examinations. Thereafter, both uterine horns were checked from cranial to caudal and in cross-section, as well as the cervices and the vagina. Then, the status of the endometrium and intra-luminal contents was evaluated. For standard evaluation of the entire reproductive tract and the assessment of ovaries, an 8–16 MHz probe was used. Depending on the reproductive state, probes with higher (early pregnancy stages) or lower frequency (late pregnancy stages) were used for better specification and exact measurement of the concepti. All measurements of organs and concepti were always taken in the same manner at the point of maximum diameter or length. The examination was completed by weighing and postanaesthetic observation if necessary. Flushing of oviducts Oviduct flushing was performed after an evaluation of a vaginal smear to confirm successful insemination with a fertile male and an ultrasonographic evaluation of the ovaries to confirm that an ovulation had occurred and successful fertilization was very likely. Six females were killed and their oviducts extracted. An intravenous catheter connected to a 10 ml syringe was cautiously inserted into the cranial part of the fallopian tube and left and right oviducts were flushed twice separately using PBS (Dulbecco's phosphate-buffered saline SIGMA 500, Sigma Aldrich Company) and a Petri dish. The flushed solution was assessed under a microscope, and embryos were counted and assessed according to their developmental stage ( Supplementary Fig. S1 , Supplementary Table S1 ). Vasectomy and genetic analysis For vasectomy ( n= 6), males were anaesthetized [11] and 1 cm of every spermatic cord removed according to general surgical principles. Paternity analyses were based on the amplification of six highly polymorphic microsatellite loci [17] , [24] using tissue samples (skin biopsy specimens from n= 19 offspring from five superfetation litters and blood samples from n= 13 adult hares): D7UTR1 [25] , Sat2, Sat3 and Sat8 [26] , OCELAMB and OCL1 [27] in experimental pairs of temporary breeders. Paternity was assessed by comparing offspring alleles with maternal alleles and the alleles of the two candidate males ( Supplementary Table S2 ). Statistical analysis Statistical calculations were performed using SPSS 15.0 statistical software (SPSS). Results are quoted as means ± s.d., and probabilities are for two-tailed tests. Statistical tests and post hoc multiple comparisons were applied following Conover [28] . The significance of Kruskal–Wallis, Wilcoxon signed-rank and Mann–Whitney U -tests was calculated with StatXact 7.0 (Cytel) and based on exact P -values for sample sizes below 30. We used GLMMs to examine factors that influenced litter size and the number of ovulations (ultrasonographically detected as the number of corpora lutea) per litter. The mode of conception (with or without superfetation) was entered as a fixed factor and maternal identity, the order of the litter in the reproductive season (first litter, second litter and so on for each female) within each year of reproduction of each female and the order of the year of reproduction (first year, second year and so on of reproduction for each female) were entered as random factors. In comparison with other conceivable analyses of longitudinal data, GLMMs have the advantage of using all data, accepting that the error structure may be correlated because of repeated measurements of the same individual, cope with variable numbers of repeats between individuals (females) and can handle the unusual problem that the fixed factor (mode of conception) did not just vary between individuals but varied both between and within individuals (and was excluded for biological reasons from being present during the first litter). Residuals of the model for the number of corpora lutea per litter did not deviate from a normal distribution (Anderson–Darling test, test statistic=0.74, P= 0.53) but did for litter size. Therefore, the variable litter size was transformed with the help of the Box-Cox transformation [29] and k , the parameter in the Box-Cox transformation, empirically determined to be 0.5 using a regression of log(residuals) against log(estimate) of the initial model. GLMMs were calculated using Systat 13.0 (Systat Software). How to cite this article: Roellig, K. et al . Superconception in mammalian pregnancy can be detected and increases reproductive output per breeding season. Nat. Commun. 1:78 doi: 10.1038/ncomms1079 (2010).